A cnidarian homologue of an insect gustatory receptor functions in developmental body patterning Insect gustatory and odorant receptors (GRs and ORs) form a superfamily of novel transmembrane proteins, which are expressed in chemosensory neurons that detect environmental stimuli. Here we identify homologues of GR s ( Gustatory receptor-like ( Grl ) genes) in genomes across Protostomia, Deuterostomia and non-Bilateria. Surprisingly, two Grls in the cnidarian Nematostella vectensis , NvecGrl1 and NvecGrl2 , are expressed early in development, in the blastula and gastrula, but not at later stages when a putative chemosensory organ forms. NvecGrl1 transcripts are detected around the aboral pole, considered the equivalent to the head-forming region of Bilateria. Morpholino-mediated knockdown of NvecGrl1 causes developmental patterning defects of this region, leading to animals lacking the apical sensory organ. A deuterostome Grl from the sea urchin Strongylocentrotus purpuratus displays similar patterns of developmental expression. These results reveal an early evolutionary origin of the insect chemosensory receptor family and raise the possibility that their ancestral role was in embryonic development. The insect chemosensory receptor superfamily, including gustatory receptors (GRs) and odorant receptors (ORs) (which represent an expanded clade within the GR family [1] ), are polytopic membrane proteins responsible for detecting a vast number of non-volatile and volatile chemicals in the environment [2] , [3] . Most sequenced insect genomes are predicted to encode several dozen to a few hundred highly divergent GRs and/or ORs [4] . Almost all of these receptors are likely to be expressed in small subsets of sensory neurons in peripheral chemosensory organs. Here they recognize external chemical cues—including esters, alcohols, ketones and volatile lipid-derived pheromones (for ORs), and sugars, bitter compounds and cuticular pheromones (for GRs)—to permit perception of food, environmental dangers, kin and potential mates [5] , [6] . A few exceptional GRs have either internal chemosensing or other sensory functions [7] , [8] , [9] . In the presence of their cognate ligands, these receptors induce neuronal firing, although their signalling mechanism is poorly understood. ORs are thought to function as odour-gated ion channels [10] , [11] , formed by a complex of an odour-specific OR and a co-receptor, ORCO [12] . GRs are less well characterized molecularly: although they are also likely to function ionotropically [13] , it remains unclear whether they function alone or in complexes of co-expressed GR subunits [14] . Understanding the molecular mechanism by which GRs and ORs act has been hampered by their lack of sequence similarity to either known ion channels or other types of membrane protein. The receptors are predicted to contain seven transmembrane domains (TMDs), similar to G protein-coupled receptors (GPCRs). Their membrane topology is, however, inverted compared with GPCRs, defining them as a distinct class of transmembrane protein [12] , [15] , [16] . Thus, despite the widespread function for insect chemosensory receptors in mediating perception of the external chemical world, the genesis of this protein family is unknown. In this work, we have used comparative genomics to characterize the evolutionary origins and dynamics of this family of receptors, and experimental analyses of GR homologues in species distant from insects to reveal an unexpected role for these proteins during embryonic development. Deep conservation of Grl genes We performed TBLASTN and PSI-BLAST searches using insect GRs and ORs as queries to identify putative homologous genes within non-insect genomes available at NCBI and other public genome and Expressed Sequence Tag (EST) databases (see Methods) ( Fig. 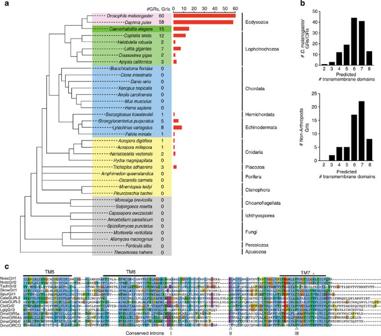Figure 1: Identification ofGrlgenes. (a) Summary of theGR/Grlrepertoires identified in the genomes of selected arthropods (pink), non-arthropod Ecdysozoa (dark green), Lophotrochozoa (light green), Deuterostomia (blue) and non-Bilateria (yellow). An unscaled tree showing the phylogenetic relationships between these species is illustrated on the left; relationships among the different non-bilaterian phyla is unresolved, with the exception of the Cnidaria, which are the closest sister group to Bilateria62. Related genes were identified in multiple species of nematode worms but, for simplicity, onlyC. elegansis shown. (b) Computational predictions of the number of TMDs found inD. melanogasterGRs and ORs (top), and Grls (bottom). Grl sequence fragments (lacking start/stop codons) were excluded from this analysis. (c) Alignment of the C-terminal regions of select insect GRs and ORs,C. elegansGURs and Grls. Predicted TMDs are indicated with horizontal lines. The asterisk marks a conserved tyrosine residue important for ion conduction in insect ORs31. The arrowheads below the alignment indicate the positions of three phase 0 ancestral GR introns (inferred from analysis ofD. melanogasterGRs and ORs1) that are conserved inGrls: intron I is conserved in phase and position inNvecGrl1,NvecGrl2,TadhGrl2,SpurGrl1,CeleGUR-2,CeleGUR-3,CtelGrl2andLgigGrl3; intron II is conserved in phase and position inNvecGrl1,NvecGrl2,TadhGrl2,SpurGrl1,CtelGrl2andLgigGrl3. Intron III is conserved in all sequences. 1a , Supplementary Table 1 and Supplementary Data 1 ). Within Protostomia, these searches recovered the previously described GRs of the crustacean Daphnia pulex (water flea) [17] , and the gustatory related ( gur ) and serpentine receptor class R ( srr ) genes of Caenorhabditis elegans [1] , [18] , [19] and other nematodes. Beyond Ecdysozoa, we identified what we term GR-like ( Grl ) genes in Lophotrochozoa, including the annelids Capitella teleta (polychaete worm) and Helobdella robusta (freshwater leech) [20] , and the molluscs, Lottia gigantea (owl limpet) [20] , Crassostrea gigas (Pacific oyster) [21] and Aplysia californica (sea slug). We also found homologous genes in Deuterostomia, including the hemichordate Saccoglossus kowalevskii (acorn worm), and several echinoderms, including the sea urchin S. purpuratus [22] , but not in any chordate ( Fig. 1a ). Finally, we identified a small number of Grl genes in non-bilaterian species, including Cnidaria, such as the sea anemone N. vectensis [23] (independently noted in another study [24] ), the corals Acropora digitifera [25] and Acropora millepora , and the placozoan Trichoplax adhaerens [26] . However, no sequences were recovered from the genomes of another cnidarian, Hydra magnipapillata , the ctenophores Mnemiopsis leidyi [27] and Pleurobrachia bachei [28] , or the sponges Amphimedon queenslandica [29] and Oscarella carmela [30] . No fungal, unicellular eukaryotic or prokaryotic genomes contained identifiable Grls ( Fig. 1a ). Figure 1: Identification of Grl genes. ( a ) Summary of the GR / Grl repertoires identified in the genomes of selected arthropods (pink), non-arthropod Ecdysozoa (dark green), Lophotrochozoa (light green), Deuterostomia (blue) and non-Bilateria (yellow). An unscaled tree showing the phylogenetic relationships between these species is illustrated on the left; relationships among the different non-bilaterian phyla is unresolved, with the exception of the Cnidaria, which are the closest sister group to Bilateria [62] . Related genes were identified in multiple species of nematode worms but, for simplicity, only C. elegans is shown. ( b ) Computational predictions of the number of TMDs found in D. melanogaster GRs and ORs (top), and Grls (bottom). Grl sequence fragments (lacking start/stop codons) were excluded from this analysis. ( c ) Alignment of the C-terminal regions of select insect GRs and ORs, C. elegans GURs and Grls. Predicted TMDs are indicated with horizontal lines. The asterisk marks a conserved tyrosine residue important for ion conduction in insect ORs [31] . The arrowheads below the alignment indicate the positions of three phase 0 ancestral GR introns (inferred from analysis of D. melanogaster GRs and ORs [1] ) that are conserved in Grls : intron I is conserved in phase and position in NvecGrl1 , NvecGrl2 , TadhGrl2 , SpurGrl1 , CeleGUR-2 , CeleGUR-3 , CtelGrl2 and LgigGrl3 ; intron II is conserved in phase and position in NvecGrl1 , NvecGrl2 , TadhGrl2 , SpurGrl1 , CtelGrl2 and LgigGrl3 . Intron III is conserved in all sequences. Full size image Several observations support the classification of the identified genes as Grl s. First, reciprocal BLAST with each Grl sequence against insect genomes identified an insect GR as the most significant hit. Second, the encoded proteins each contain multiple predicted TMDs—most commonly 6–7 TMDs in putative full-length Grl sequences—similar to GRs and ORs ( Fig. 1b ). (Accurate computational predictions of TMD number and topology are difficult because of the variable hydrophobicity of TMDs within this family of receptors [12] ). Third, the phase and position of three inferred ancestral introns in the 3′ region of Drosophila melanogaster GR transcripts [1] are well-conserved in Grls ( Fig. 1c ). Finally, Grls share a number of characteristic amino acid residues with the most highly conserved C-terminal region of the insect receptors, including a tyrosine residue important for ion channel function in insect ORs [31] ( Fig. 1c ). The overall sequence similarity of Grls and insect GRs (or ORs) is very low (~15%–20% amino acid identity, similar to the minimum identity within the GR and OR families themselves [1] ), with the highest similarity to the GR64a-f/GR61a clade of sugar-sensing receptors [14] . Phylogenetic analysis revealed no unambiguous orthologous relationships of Grls with any insect GR, or between Grls of different lophotrochozoan, deuterostome or non-bilaterian species ( Fig. 2 ). Although the high divergence of these sequences precludes accurate reconstruction of their ancestry, many members of these repertoires appear to have formed by species-specific expansions ( Fig. 2 ). 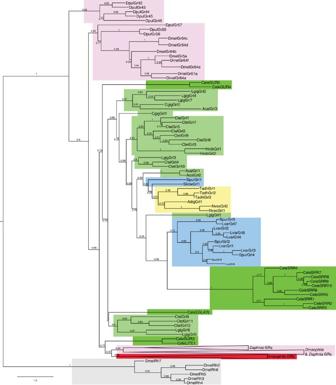Figure 2: Phylogenetic analysis of Grl, GR and OR genes. Maximum likelihood tree showing the relationships between select arthropod GRs/ORs,C. elegansGURs and all Grls (except the short sequence fragments predicted inP. miniataandA. millepora), colour coded as inFig. 1a.DrosophilaRhodopsins are included as an outgroup; although it remains unclear whether these two different families of heptahelical membrane proteins share a common ancestor, they clearly belong to a separate clade. For clarity, branches for large clades ofD. melanogasterGRs/ORs orD. pulexGRs have been collapsed. The scale bar represents the number of amino acid substitutions per site. Figure 2: Phylogenetic analysis of Grl, GR and OR genes. Maximum likelihood tree showing the relationships between select arthropod GRs/ORs, C. elegans GURs and all Grls (except the short sequence fragments predicted in P. miniata and A. millepora ), colour coded as in Fig. 1a . Drosophila Rhodopsins are included as an outgroup; although it remains unclear whether these two different families of heptahelical membrane proteins share a common ancestor, they clearly belong to a separate clade. For clarity, branches for large clades of D. melanogaster GRs/ORs or D. pulex GRs have been collapsed. The scale bar represents the number of amino acid substitutions per site. Full size image Early developmental expression of Grl genes in N. vectensis To investigate the role of Grls in non-Arthropoda, we focused in this study on the cnidarian N. vectensis (here abbreviated Nvec ), which is amenable to gene expression and functional analyses. Moreover, the development and anatomy of this organism are relatively well-described, and a presumed chemosensory structure, the apical organ, has been identified ( Fig. 3a ) [32] , [33] . N. vectensis development proceeds through a coeloblastula stage to gastrulation, which occurs mainly by invagination [34] , [35] . After gastrulation, the embryo emerges from the egg jelly as a free-swimming planula, which moves by ciliary beating with the apical sense organ pointing forward. Subsequently, the planula transforms (‘metamorphoses’) into a sessile polyp, which starts feeding after formation of the tentacles that surround the single opening of the animal ( Fig. 3a ). 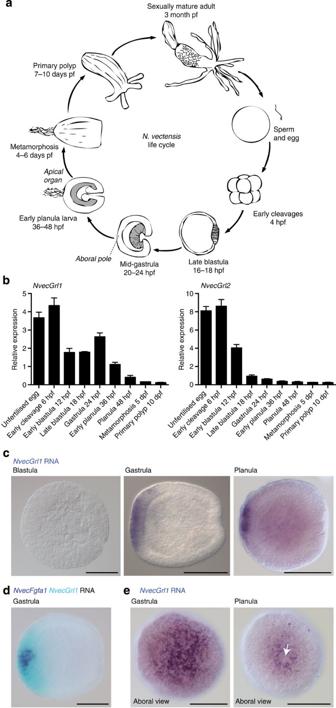Figure 3:N. vectensisGrls are expressed during early development. (a) Schematic of the life cycle of the sea anemoneN. vectensis. Dark grey shading in the blastula, gastrula and early planula stages indicates the endoderm. Different stages are not drawn to scale; hpf=hours post-fertilisation. (b) Quantitative reverse transcriptase–PCR analysis of the temporal expression ofNvecGrl1andNvecGrl2during nine developmental time points. Data from three biological replicate samples (mean±s.e.m.) are shown. (c) RNA in situ hybridization using a riboprobe againstNvecGrl1on whole-mountN. vectensisat three developmental stages. Lateral views, with the aboral side on the left, are shown for all specimens in this and subsequent figures, unless otherwise noted. (d) Two-colour RNA in situ hybridization using riboprobes againstNvecGrl1(light blue) andNvecFgfa1 (dark blue) on whole-mountN. vectensisembryos. (e) RNA in situ hybridization using a riboprobe againstNvecGrl1on whole-mountN. vectensisat two developmental stages showing an aboral view, which reveal the formation of a ring-like distribution of transcripts at the planula stage. The apical organ forms from the unstained cells inside the ring (white arrow). Scale bars, 100 μm (c–e). Figure 3: N. vectensis Grls are expressed during early development. ( a ) Schematic of the life cycle of the sea anemone N. vectensis . Dark grey shading in the blastula, gastrula and early planula stages indicates the endoderm. Different stages are not drawn to scale; hpf=hours post-fertilisation. ( b ) Quantitative reverse transcriptase–PCR analysis of the temporal expression of NvecGrl1 and NvecGrl2 during nine developmental time points. Data from three biological replicate samples (mean±s.e.m.) are shown. ( c ) RNA in situ hybridization using a riboprobe against NvecGrl1 on whole-mount N. vectensis at three developmental stages. Lateral views, with the aboral side on the left, are shown for all specimens in this and subsequent figures, unless otherwise noted. ( d ) Two-colour RNA in situ hybridization using riboprobes against NvecGrl1 (light blue) and Nvec Fgfa1 (dark blue) on whole-mount N. vectensis embryos. ( e ) RNA in situ hybridization using a riboprobe against NvecGrl1 on whole-mount N. vectensis at two developmental stages showing an aboral view, which reveal the formation of a ring-like distribution of transcripts at the planula stage. The apical organ forms from the unstained cells inside the ring (white arrow). Scale bars, 100 μm ( c – e ). Full size image Surprisingly, analysis of the temporal pattern of expression of the two Grls we found in this species, NvecGrl1 and NvecGrl2 , by quantitative reverse transcriptase–PCR (qPCR) revealed the highest level of expression of these genes in early developmental stages ( Fig. 3b and Supplementary Table 2 ): NvecGrl1 is expressed in the egg and blastula, gastrula and early planula stages, diminishing rapidly to very low levels later in development ( Supplementary Table 2 ). NvecGrl2 is only robustly detected in the egg and blastula. These temporal expression profiles contrast markedly with those of D. melanogaster GRs and ORs, where expression of these receptors has been reported only in differentiated sensory neurons [5] . We next examined the spatial distribution of N. vectensis Grl transcripts by whole-mount RNA in situ hybridization on a range of developmental stages. Although NvecGrl2 RNA was undetectable in these experiments ( Supplementary Fig. 1 ), we first observed NvecGrl1 transcripts in a broad aboral domain at the gastrula stage ( Fig. 3c ). This domain develops under the control of genes homologous to those that regulate anterior (or apical) development in bilaterians [36] , and its centre is the site of formation of the apical sensory organ in the planula larva ( Fig. 3a ). Genes with similarly broad aboral expression at the gastrula stage display different expression dynamics after gastrulation: ‘spot genes’ (for example, NvecFgfa1 , NvecFgfa2 and NvecSoxB1 ) become restricted to a small spot at the aboral pole, from which the apical organ develops, whereas ‘ring genes’ (for example, NvecSix3/6 and NvecFoxQ2a ) remain expressed in a ring-like domain around the apical organ [36] . Comparison of the spatial distribution of NvecGrl1 with NvecFGFa1 by double RNA in situ hybridization revealed that the NvecGrl1 expression domain remains broad at late gastrula/early planula stages when NvecFgfa1 has already restricted to a small aboral spot ( Fig. 3d ). Subsequently, NvecGrl1 transcripts are excluded from the apical organ-forming spot ( Fig. 3e ), similar to other ‘ring genes’. Although the ‘ring gene’ domain includes some scattered sensory cells [37] , [38] , the broad and early expression of NvecGrl1 in the aboral domain indicates that this receptor may primarily have a non-chemosensory role in this species. Regulation of NvecGrl1 by the aboral patterning network Several transcription factors and signalling molecules that are expressed in the aboral region and required for apical organ formation in N. vectensis have been identified [36] . For example, the homeodomain transcription factor NvecSix3/6 is an important determinant of the aboral territory, where it initiates an autoregulatory loop of fibroblast growth factor (FGF) signalling to pattern this domain [36] . To determine whether NvecGrl1 aboral expression is regulated by these factors, we performed RNA in situ hybridization on embryos injected with morpholino oligonucleotides (morphants) designed to block translation of these genes. In NvecSix3/6 morphants, NvecGrl1 aboral expression is reduced or absent in gastrula embryos compared with control morphants, similar to other markers of this domain [36] ( Fig. 4a ), suggesting that NvecGrl1 functions downstream of this transcription factor. 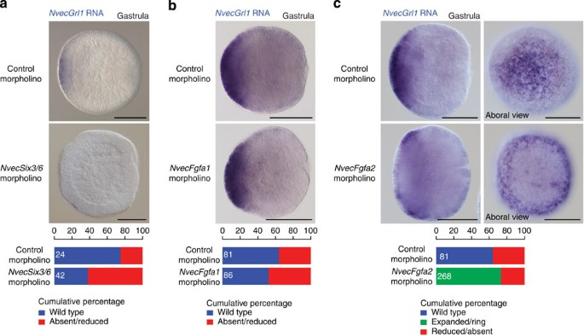Figure 4: Regulation ofN. vectensisGrl1 expression by the apical patterning network. (a) RNA in situ hybridization using a riboprobe againstNvecGrl1on whole-mountN. vectensisembryos injected with either control orNvecSix3/6morpholino oligonucleotides. Quantification of the phenotypes is shown below. Note thatNvecGrl1transcripts are relatively weakly detected and a fraction of control morpholino-injected animals did not exhibit staining. Thenis shown in white within each bar in this and all equivalent graphs. (b) RNA in situ hybridization using a riboprobe againstNvecGrl1on whole-mountN. vectensisembryos injected with either control orNvecFgfa1morpholino oligonucleotides. Quantification of the phenotypes is shown below. (c) RNA in situ hybridization using a riboprobe againstNvecGrl1on whole-mountN. vectensisembryos injected with either control orNvecFgfa2morpholino oligonucleotides. InNvecFgfa2morphants, note the precocious formation and larger size of the ring ofNvecGrl1transcripts around the aboral pole (compare withFig. 3e). Quantification of the phenotypes is shown below. Scale bars, 100 μm (a–c). Figure 4: Regulation of N. vectensis Grl1 expression by the apical patterning network. ( a ) RNA in situ hybridization using a riboprobe against NvecGrl1 on whole-mount N. vectensis embryos injected with either control or NvecSix3/6 morpholino oligonucleotides. Quantification of the phenotypes is shown below. Note that NvecGrl1 transcripts are relatively weakly detected and a fraction of control morpholino-injected animals did not exhibit staining. The n is shown in white within each bar in this and all equivalent graphs. ( b ) RNA in situ hybridization using a riboprobe against NvecGrl1 on whole-mount N. vectensis embryos injected with either control or NvecFgfa1 morpholino oligonucleotides. Quantification of the phenotypes is shown below. ( c ) RNA in situ hybridization using a riboprobe against NvecGrl1 on whole-mount N. vectensis embryos injected with either control or NvecFgfa2 morpholino oligonucleotides. In NvecFgfa2 morphants, note the precocious formation and larger size of the ring of NvecGrl1 transcripts around the aboral pole (compare with Fig. 3e ). Quantification of the phenotypes is shown below. Scale bars, 100 μm ( a – c ). Full size image NvecFgfa1 and NvecFgfa2 participate in positive and negative feedback regulation of apical organ formation, respectively [33] , [36] : NvecFgfa1 morphants fail to develop an apical organ [33] , whereas NvecFgfa2 morphants display precocious formation of an expanded apical organ [36] . However, although effects of NvecFgfa1 knockdown become visible only after gastrulation, an expansion and/or upregulation of apical organ domain genes in NvecFgfa2 knockdown animals is detectable already at gastrula stage [36] . Consistently, we found that the expression of NvecGrl1 appears only slightly affected in NvecFgfa1 morphants at the end of gastrulation ( Fig. 4b ). By contrast, in NvecFgfa2 morphants, NvecGrl1 expression forms an expanded ring with a wider area of low NvecGrl1 expression in its centre and this ring-like domain appears earlier than in control animals ( Fig. 4c compared with Fig. 3e ). These data provide further evidence that NvecGrl1 is expressed in cells that do not directly give rise to the apical sensory organ. Grl1 is required for aboral patterning in N. vectensis To investigate the function of NvecGrl1 , we injected zygotes with morpholino oligonucleotides designed to block translation of this receptor, and examined development of these animals in parallel with those injected with control morpholinos (see Methods). Early developmental processes, including gastrulation, appeared to proceed normally in both NvecGrl1 and control morphant animals ( Fig. 5a ). However, NvecGrl1 morphants displayed pronounced morphological defects in the apical organ domain in planula larvae ( Fig. 5a,b ). In control animals, the first sign of apical organ formation is the translocation of the nuclei in a small group of cells at the aboral pole to a more basal position ( Fig. 5a ). These cells subsequently form a small indentation of the aboral ectoderm ( Fig. 5a ); this indentation is the site from which the long cilia of the apical organ emerge [37] . In NvecGrl1 morphants, the initial basal movement of nuclei is absent or strongly reduced, and no clear indentation develops ( Fig. 5a ). Correspondingly, the apical tuft is absent or consists of only few long cilia in 4-day-old NvecGrl1 morphants ( Fig. 5b ). These animals subsequently fail to develop into primary polyps (0%, n =159 NvecGrl1 morphants, compared with control morphants 63%, n =122). These defects were reproduced with a second morpholino against NvecGrl1 (<9% primary polyps, n =109). 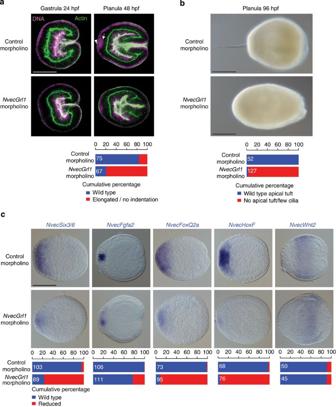Figure 5:N. vectensisGrl1 is required for aboral pole patterning. (a) Morphological phenotypes ofN. vectensisembryos injected with either control (control#1) orNvecGrl1(NvecGrl1#1) morpholino oligonucleotides, in which DNA (magenta) and the actin cytoskeleton (green) are labelled with TO-PRO-3 and Alexa Fluor 488 Phalloidin, respectively. The arrow marks the group of nuclei at the aboral pole that have translocated to a more basal position (towards the right of the image) in control but notNvecGrl1morphants; this results in these cells forming a small indentation of the apical ectoderm (arrowhead). Scale bar, 100 μm (applies to all images). Quantification of the phenotypes is shown below. (b) Bright-field images of living 4-day planulae derived fromN. vectensisembryos injected with either control (control#1) orNvecGrl1(NvecGrl1#2) morpholino oligonucleotides revealing the failure in apical tuft develops inNvecGrl1morphants. Quantification of the phenotypes is shown below. Scale bars, 100 μm. (c) RNA in situ hybridization using probes against marker genes in animals injected with either control (control#1) orNvecGrl1(NvecGrl1#1) morpholino oligonucleotides. Scale bar, 100 μm (applies to all images). Quantification of the phenotypes is shown below. Figure 5: N. vectensis Grl1 is required for aboral pole patterning. ( a ) Morphological phenotypes of N. vectensis embryos injected with either control (control#1) or NvecGrl1 ( NvecGrl1#1 ) morpholino oligonucleotides, in which DNA (magenta) and the actin cytoskeleton (green) are labelled with TO-PRO-3 and Alexa Fluor 488 Phalloidin, respectively. The arrow marks the group of nuclei at the aboral pole that have translocated to a more basal position (towards the right of the image) in control but not NvecGrl1 morphants; this results in these cells forming a small indentation of the apical ectoderm (arrowhead). Scale bar, 100 μm (applies to all images). Quantification of the phenotypes is shown below. ( b ) Bright-field images of living 4-day planulae derived from N. vectensis embryos injected with either control (control#1) or NvecGrl1 ( NvecGrl1#2 ) morpholino oligonucleotides revealing the failure in apical tuft develops in NvecGrl1 morphants. Quantification of the phenotypes is shown below. Scale bars, 100 μm. ( c ) RNA in situ hybridization using probes against marker genes in animals injected with either control (control#1) or NvecGrl1 ( NvecGrl1#1 ) morpholino oligonucleotides. Scale bar, 100 μm (applies to all images). Quantification of the phenotypes is shown below. Full size image To understand the basis for these morphological defects, we analysed expression of aboral domain patterning genes in NvecGrl1 morphants. NvecSix3/6 expression is greatly diminished—but not abolished—in NvecGrl1 morphants at the planula stage compared with control morphants ( Fig. 5c ). Consistent with the reduction of NvecSix3/6 expression, two of its downstream targets, the transcription factor NvecFoxQ2a and NvecFgfa2 (ref. 36 ), are also reduced in NvecGrl1 morphants compared with controls ( Fig. 5c ). Defects in gene expression were also detectable at gastrula stages ( Supplementary Fig. 2a ), when NvecGrl1 transcripts are first detected in the aboral domain, although these phenotypes were very subtle, though consistent, for NvecSix3/6 and NvecFoxQ2a . Together, these observations implicate NvecGrl1 in a feedback pathway that maintains NvecSix3/6 expression to pattern the aboral domain. By contrast, patterning genes expressed elsewhere in the embryo, for example, NvecWnt2 , which is found in a belt-like domain between the aboral and oral poles [39] , are not or at most mildly affected in NvecGrl1 morphants ( Fig. 5c ). One of the important functions of the FGF signalling loop is to downregulate NvecSix3/6 expression after gastrulation in a small ‘spot’, the developing apical organ domain. Within this spot, genes required for apical organ formation, such as the transcription factor NvecHoxF , are expressed [36] . Defects in the initiation of FGF signalling leads to a failure in formation of this NvecSix3/6 -and NvecFoxQ2a -negative and NvecHoxF -positive aboral spot [36] . We observed a similar phenotype in NvecGrl1 , but not control, morphants ( Fig. 5c and Supplementary Fig. 2b ); these defects could account for failure of apical organ development. Together, these results support a role for NvecGrl1 in the regulatory network that controls aboral domain patterning and thereby apical sensory organ formation. Developmental expression of a deuterostome Grl gene To determine whether the early developmental expression of Grl genes is conserved in Deuterostomia, we used qPCR to analyse transcript levels of the five Grls of the echinoderm S. purpuratus during embryonic stages ( Fig. 6a ). Notably, SpurGrl1 , which is the most similar sea urchin Grl to NvecGrl1 ( Fig. 2 ), was detected during early development ( Fig. 6b and Supplementary Table 3 ): the highest expression of SpurGrl1 was at the blastula stage, but it remained at elevated levels in the gastrula and later embryonic developmental stages. These qPCR data are in agreement with quantitative developmental transcriptome data ( Supplementary Fig. 3a ) [40] . The other four SpurGrls were expressed at only very low levels during developmental stages ( Fig. 6b ), but transcripts could be readily amplified for all SpurGrls , except SpurGrl3 , from adult neural tissue ( Supplementary Fig. 3b ). These observations suggest that SpurGrl1 has a unique function during embryonic development. 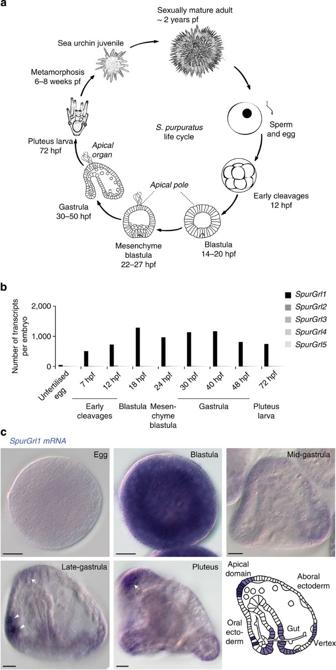Figure 6: Early developmental expression of anS. purpuratusGrl. (a) Schematic of the life cycle of the sea urchinS. purpuratus. (b) Quantitative reverse transcriptase–PCR analysis of the temporal expression of the fiveSpurGrlgenes during nine developmental time points. Data are represented as number of transcripts per embryo and represent the average of four technical replicates in each of two independent biological replicate samples (seeSupplementary Table 3). (c) RNA in situ hybridization using a riboprobe againstSpurGrl1on whole-mountS. purpuratusof five developmental stages. All the embryos represent lateral views: as indicated in the schematic, the oral ectoderm is on the left and the apical domain on the top in the gastrula and pluteus specimens. The arrows mark the expression ofSpurGrl1in the apical domain (where the apical organ will form), while the arrowheads mark a pair of presumptive neurosecretory cells in the oral ectoderm. Scale bars, 20 μm. Figure 6: Early developmental expression of an S. purpuratus Grl. ( a ) Schematic of the life cycle of the sea urchin S. purpuratus . ( b ) Quantitative reverse transcriptase–PCR analysis of the temporal expression of the five SpurGrl genes during nine developmental time points. Data are represented as number of transcripts per embryo and represent the average of four technical replicates in each of two independent biological replicate samples (see Supplementary Table 3 ). ( c ) RNA in situ hybridization using a riboprobe against SpurGrl1 on whole-mount S. purpuratus of five developmental stages. All the embryos represent lateral views: as indicated in the schematic, the oral ectoderm is on the left and the apical domain on the top in the gastrula and pluteus specimens. The arrows mark the expression of SpurGrl1 in the apical domain (where the apical organ will form), while the arrowheads mark a pair of presumptive neurosecretory cells in the oral ectoderm. Scale bars, 20 μm. Full size image By whole-mount RNA in situ hybridization, we observed that SpurGrl1 exhibits a dynamic spatial expression pattern during early development ( Fig. 6c ). In the blastula SpurGrl1 RNA was present ubiquitously, while in later stages it was restricted to a few groups of cells. From the late gastrula, transcripts were detected in cells in the apical domain, which develops into a neurosensory structure [41] . Strong SpurGrl1 expression was also detected in two bilaterally arrayed cells in the oral ectoderm and, at lower levels, in the hindgut and adjacent ectoderm, as well as a region of the aboral ectoderm that will develop into the vertex ( Fig. 6c ). The apical domain expression of SpurGrl1 represents an intriguing parallel with that of NvecGrl1 in the developmentally equivalent region of the sea anemone gastrula [36] , [42] , [43] , although the additional expression patterns suggest that the sea urchin gene has several functions. We have defined an early evolutionary origin and broad phylogenetic distribution of the insect chemosensory receptor superfamily. Previously only characterized in Ecdysozoa [2] , [17] , [44] , [45] , we show Grl genes are present in genomes across Protostomia, non-chordate Deuterostomia and non-Bilateria. These observations establish the origin of this gene family before the split of Bilateria and non-Bilateria 550–850 million years ago [46] , and suggest that these genes have been lost in the ancestral chordate. Through analysis of Grls in the non-bilaterian N. vectensis , we found—unexpectedly—several lines of evidence supporting a role in developmental body patterning rather than external chemosensation. First, the existence of a small number of NvecGrls is inconsistent with this cnidarian receptor repertoire playing a wide-ranging role in the detection of environmental chemical signals. We note that N. vectensis has several dozen vertebrate OR-like GPCRs, which represent candidate chemosensory receptors of this species [47] . Second, in contrast to Drosophila ORs and GRs [48] , both NvecGrl s are expressed in early developmental stages, before formation of sensory neurons and a putative chemosensory organ (at late gastrula and mid-planula stage, respectively [37] , [38] ). Moreover, NvecGrl1 transcripts are detected broadly around the aboral pole in gastrula and planula stages, but are selectively excluded from an aboral ‘spot’ of cells that subsequently gives rise to the apical sensory organ. Third, functional analysis of NvecGrl1 supports a role in aboral body patterning essential for developmental progression. Although our data argue that NvecGrls have a different function to insect GRs, we cannot exclude that they have a later, additional role, for example, in the detection of metamorphosis-related sensory signals. Although loss of NvecGrl1 blocks developmental progression beyond the planula stage, the relatively limited current knowledge of aboral patterning in Cnidaria makes it difficult to define the precise role of this protein. Our data are consistent with a model in which NvecGrl1 functions downstream of the aboral territory determinant NvecSix3/6 in the feedback loop that is important to refine aboral pole patterning and promote apical organ formation [36] . Secondary structure and sequence conservation of NvecGrl1 (and other Grls) with insect GRs and ORs suggest that this protein acts as a ligand-gated ion channel and might recognize a paracrine developmental signal; testing this model will require identification of a relevant ligand. Nevertheless, it is intriguing that NvecGrl1 plays a role in the formation (albeit indirectly) rather than the function of a putative chemosensory organ. We have not been able detect transcripts for NvecGrl2 gene in situ and morpholino-mediated knockdown of NvecGrl2 did not reveal any obvious patterning defects (unpublished data), suggesting that this gene has a different role to NvecGrl1 . The similarities in the early developmental expression of the deuterostome Grl gene with highest sequence identity to NvecGrl1 , S. purpuratus Grl1 , hints that a role in embryonic patterning may have been an ancestral function of this family. However, SpurGrl1 displays additional spatial expression patterns beyond the apical domain and four additional SpurGrls do not show such early expression, suggesting that Grls in this species have multiple different roles. Cleanly dissecting the function of SpurGrl1 (and its paralogues) will require methods that permit tissue-specific gene knockdown. Beyond the work presented here, very little is known about the role of members of the GR/Grl family outside insects. The large size and high sequence divergence of the GR repertoire in the crustacean D. pulex is consistent with a role in chemosensation [17] , although no expression or functional analyses of these receptors have been reported. The nematode C. elegans relies on a very large family of GPCRs for chemical detection [18] , and of the 15 Grl genes (the gur and srr families [1] , [18] , [19] , the latter not previously defined as members of this superfamily) only two have been characterized. GUR-2 (also known as LITE-1) functions in photosensitive neurons [44] , [45] , although it has not been determined whether this protein senses light directly. GUR-1 (also known as EGL-47) appears to regulate motoneurons that control egg laying [49] . Together with our data in N. vectensis and S. purpuratus , these observations suggest that Grl/GR genes may have been recruited only in arthropods to fulfil a predominant role in peripheral chemosensation. Future analysis of other Grls in a range of species should yield insights into the diverse functions and evolutionary history of this unusual receptor family. Gene identification To identify homologues of insect chemoreceptors, all known Drosophila sequences of GRs and ORs were used as queries in extensive TBLASTN and PSI-BLAST searches of public genome and EST data sets (see Supplementary Table 1 and Supplementary Data 1 ), and in screens of OrthoDB [50] . Identified genes were used in iterative BLAST searches of species-specific data sets until no new sequences were identified. The numbers of genes in most species are likely to represent minimum estimates due to the challenge of identifying highly divergent Grl genes from incompletely assembled genomes with computational predictions alone. For the same reasons, most predicted sequences are incomplete, particularly at the more divergent 5′ end. Analysis of the membrane topology (excluding partial protein sequences) was performed using TMHMM v.2.0 (ref. 51 ). Intron positions and phases were predicted by comparing cloned (or predicted) transcript sequences and the corresponding genomic sequences. Alignment/phylogenetic tree building Protein alignments were built using Clustal Omega [52] with the following settings—max HMM Iterations: 5; combined iterations: 5; max guide iterations: 5. The amino termini of the sequences were cut off after aligning using Jalview [53] and only the carboxy-terminal regions from TMD5 (starting with position 352 in DmelORCO) was used for further analysis. Tree reconstruction was performed using PhyML3.0 (ref. 54 ) and the LG model [55] was used as a substitution matrix. Branch support was calculated using the approximate likelihood-ratio test method [56] . The tree was rooted on the Rhodopsin branch, although we acknowledge that the evolutionary relationship between these receptor families is still unclear. Cloning of full-length Grl coding sequences To obtain the complete coding sequence of NvecGrl1 , PCR was performed on mixed embryo stage complementary DNA, with specific primers based on EST and genome data ( genome.jgi-psf.org/Nemve1/Nemve1.home.html ). For NvecGrl2 5′ and 3′ rapid amplification of cDNA end (RACE) PCRs were performed. The following primer sets were used: NvecGrl1 . 5′- GTGTGAGCACGCTGCGAGAATGG -3′ 3′- TCACTTAAACTGGACAAGAATCG -5′ NvecGrl2 . 5′RACE outer primer: 5′- AGAGCAGAAGGCTCACAAGC -3′ 5′RACE inner primer: 5′- CAAGGAATTTCATTGCGACAG -3′ 3′RACE outer primer: 5′- CGATTGGAGGAATTGTCCCAGTAACACGCGG -3′ 3′RACE inner primer: 5′- TCAACACAGAAGTGATCAGCCCAACGATTGG -3′ Genbank accession numbers are: KP294348 ( NvecGrl1 ) and KP294349 ( NvecGrl2 ). For SpurGrl1 , a 1,212 bp fragment of the coding sequence was amplified by PCR from 18 hpf embryonic cDNA, cloned into pGEM-T Easy (Promega) and sequenced, using the following primers designed on the WHL22.291934 transcriptome sequence: 5′- GAACACCACTCCATGGAACC -3′ 3′- CTATGGGATCACCGCTCACT -5′ Quantitative PCR For N. vectensis , cell lysates of embryonic stages were collected and total RNA was extracted using the RNAqueous kit (Ambion). cDNA synthesis was performed using the SuperScript II RT Reagent Kit, according to the manufacturer’s protocol. Expression of NvecGrl1 , NvecGrl2 and reference genes were analysed by performing PCR on an Applied Biosystems 7900HT SDS, using the cDNA as template and SYBR Premix (Roche) with the following primers: NvecGrl1 5′- AATCGTGCTAGCCACATTCTGGTG -3′ 3′- ACCTCGTACACAACGCCTGTCAAA -5′ NvecGrl2 5′- ACTATAGTAACGTCACTTGCGGGTGC -3′ 3′- TTCGCCGTCTTTCAGTTCATCCAC -5′ Ef1b 5′- TGCTGCATCAGAACAGAAACCTGC -3′ 3′- TAAGCCTTCAAGCGTTCTTGCCTG -5′ RibPrL23 5′- TTACGGAGCTCTGGCTTTCCTTTC -3′ 3′- TGCCGTTAAGGGTATCAAAGGACG -5′ The reference target stability values were as follows EF1α ( M =0.404; CV=0.135), RibPr23L ( M =0.404; C =0.144), average ( M =0.404; CV=0.140). For S. purpuratus , cell lysates of appropriately staged embryos were collected and total RNA was extracted using the RNeasy Micro Kit (Qiagen). cDNA synthesis was performed using the iScript cDNA Synthesis Kit (Bio-Rad), according to the manufacturer’s instructions. At least four technical replicas were run on two independent cDNA batches, using cDNA equivalent to 1 embryo per reaction (2.8 ng) and Power SYBR Green QPCR master mix (Applied Biosystems), on the 7900HT Fast Real-Time PCR system and the following primers ( SpurUbq was used as internal standard [57] , [58] ): SpurGrl1 5′- TCTGCGAATCGAGAAGTCCT -3′ 3′ GAGCCATAGTCGCGTAGGTC -5′ SpurGrl2 5′- CATCCACGGTCTGAAGACAA -3′ 3′- GCAACTTGAAACGCCCATAC -5′ SpurGrl3 5′- GCCTCAATTTAGCGGCAGTA -3′ 3′- CCAGATAGGATGTGGCAGGT -5′ SpurGrl4 5′- ATCCTCAGCCCTTTCTGACA -3′ 3′- GAACTGGTCGGTCAGGATGT -5′ SpurGrl5 5′- ATAACGCTGAGCCGGTACAA -3′ 3′- TGGTTGCAGCAGTTTGAAAG -5′ SpurUbq 5′- CACAGGCAAGACCATCACAC -3′ 3′- GAGAGAGTGCGACCATCCTC -5′ Morpholinos Translation-blocking antisense morpholino oligonucleotides (GeneTools, LLC) were designed to match the sequence of NvecGrl1 . The sequences of the morpholinos used are: NvecGrl1#1 : 5′- ACGCTCCGACTGGAACTGC CAT TCA -3′ NvecGrl1#2 : 5′- GAACTGC CAT TCATTCCGCTTGTTC -3′ control#1 (generic [36] ): 5′- CCATTGTGAAGTTAAACGATAGATC -3′ control#2 ( NvecGrl1 mismatch): 5′- ACGCGCCTACTGGAATTGCTATTAA -3′ The two morpholinos against NvecGrl1 are partially overlapping to avoid 5′-untranslated region sequence that is present elsewhere in the genome. The sequence corresponding to the start codon in the NvecGrl1 morpholinos is underlined. Six3/6 : 5′- GTACTGCCGCACTGCAAGACTTGTC -3′ (ref. 36 ) Fgfa1 : 5′- ATAAGGTGGACGCATGACTTTGTAG -3′ Fgfa2 : 5′- CGTTAGCATGGTGATCGTCATGTTG -3′ (ref. 33 ) Nematostella culture, manipulation and microinjection Animals were cultured at 18 °C in 1:3 diluted sea water in the Sars Centre Cnidaria facility, and gamete production was induced by overnight exposure to light and elevated temperature (25 °C) [59] . Morpholinos were diluted in H 2 O, together with a tracer (Alexa568 Dextran (Molecular Probes) at 0.1 mg ml −1 ), to a final concentration of either 1 mM ( NvecGrl1 #1) or 0.6 mM ( NvecGrl1 #2); control morpholinos were diluted to the same concentration in parallel experiments. Zygotes were microinjected using an Eppendorf Femtojet, with a volume equivalent to ~5% of the egg. Following injections, the embryos were transferred to Petri dishes containing Nematostella medium and were allowed to develop at 21 °C until fixation. For images of live planulae, animals were mounted in 2% methylcellulose (in Nematostella medium) and imaged on a Nikon Eclipse E800 microscope. Histology N. vectensis . For actin and DNA staining, specimens were fixed in 4% formaldehyde in PBT (0.1% Triton X-100 in PBS) for 1 h and washed four times in PBT. 30 μl of Alexa Fluor 488 Phalloidin (Molecular Probes) were put in an open Eppendorf tube for 30 min at room temperature, to let the solvent evaporate. The pellet was redissolved in 1.5 ml PBT and 1.5 μl TO-PRO-3 Iodide (Molecular Probes) was added. The specimens were incubated for 2–3 h in this staining solution, washed five times with PBT and mounted in ProLong Gold (Life Technologies). RNA in situ hybridization on N. vectensis was performed using antisense digoxygenin-labelled probes against the open reading frame (ORF) of the desired genes essentially as described [60] . In brief, hybridization was carried out at 60 °C for 60 h, and post-hybridization stringency washes were with 0.01 × SSCT. Anti-digoxygenin Fab fragments (Roche) were diluted 1:5,000 before detection by NBT/BCIP staining (Roche). For N. vectensis double in situ hybridization, digoxygenin-labelled NvecGrl1 and fluorescein isothiocyanate-labelled NvecFgfa1 probes complementary to the corresponding ORF were used. NvecFgfa1 was detected by NBT/BCIP staining and NvecGrl1 was detected using anti-DIG-POD and tyramide-based signal amplification (TSA plus DNP (AP) kit, Perkin Elmer), followed by anti-DNP-AP-mediated BCIP staining. S. purpuratus . Specimens were fixed in 4% formaldehyde in MOPS buffer overnight at 4 °C, then washed several times in MOPS buffer and once in 70% ethanol. After rehydration in TBST, RNA in situ hybridization was performed using an antisense digoxygenin-labelled probe against the 1,212 bp fragment of the SpurGrl1 ORF (see above) as described [61] . In brief, 0.05 ng μl −1 of probe was hybridized at 60 °C for 16 h. Post-hybridization stringency washes were with 0.1 × SSC and 0.01 × SSC. Anti-digoxygenin Fab fragments were diluted 1:2,000 before detection by NBT/BCIP staining. How to cite this article : Saina, M. et al . A cnidarian homologue of an insect gustatory receptor functions in developmental body patterning. Nat. Commun. 6:6243 doi: 10.1038/ncomms7243 (2015).